Atomically-precise colloidal nanoparticles of cerium dioxide Synthesis of truly monodisperse nanoparticles and their structural characterization to atomic precision are important challenges in nanoscience. Success has recently been achieved for metal nanoparticles, particularly Au, with diameters up to 3 nm, the size regime referred to as nanoclusters. In contrast, families of atomically precise metal oxide nanoparticles are currently lacking, but would have a major impact since metal oxides are of widespread importance for their magnetic, catalytic and other properties. One such material is colloidal CeO 2 (ceria), whose applications include catalysis, new energy technologies, photochemistry, and medicine, among others. Here we report a family of atomically precise ceria nanoclusters with ultra-small dimensions up to ~1.6 nm (~100 core atoms). X-ray crystallography confirms they have the fluorite structure of bulk CeO 2 , and identifies surface features, H + binding sites, Ce 3+ locations, and O vacancies on (100) facets. Monodisperse ceria nanoclusters now permit investigation of their properties as a function of exact size, surface morphology, and Ce 3+ :Ce 4+ composition. Since its introduction in 1976 as an oxygen-storage component to ensure the efficient activity of the noble metals used in three-way catalysis in automobile exhausts [1] , [2] , [3] , cerium(IV) dioxide (CeO 2 , ceria) has become of considerable utility as a catalyst or co-catalyst in industrial, petrochemical and environmental processes [2] , [3] , [4] , [5] , [6] , [7] . In addition, CeO 2 -containing materials are often used in oxide fuel cells [8] , precision polishing materials [9] , [10] , UV filters [10] , corrosion prevention [11] , and other applications [1] , [12] , [13] .This widespread use of Ce is partially due to its significant abundance (0.0046% by weight of the Earth’s crust) and its Ce 3+ /Ce 4+ redox couple, which is crucial to many applications by facilitating the formation of CeO 2− x , containing highly reactive defect sites comprising O vacancies and attendant Ce 3+ ions [1] , [12] , [14] . Ceria can thus act as an efficient oxygen buffer, assisted by oxygen mobility within its layered fluorite structure. In fact, bulk ceria naturally contains relatively few Ce 3+ /O-vacancy defect sites at ambient temperatures, but their number increases at higher temperatures where Ce 4+ reduction and oxygen release are favoured. Catalysis by bulk ceria is therefore normally carried out at temperatures > 450 °C. In the last decade, interest in ceria nanoparticles (CNPs) has seen explosive growth due to their much greater reactivity and increased catalytic efficiencies at lower temperatures [9] , [12] . Significant CNP activity at or near room temperature has also been established [15] , as has facet-dependent reactivity [12] , [16] . For example, appreciable oxygen storage capacity is observed at 150 °C on the cubic (100) face of nanoceria crystals, which is ~250 °C lower than for irregularly shaped nanoceria or the bulk material [17] . CNPs are also under investigation as photovoltaic materials in solar cells whereas bulk CeO 2 has no photovoltaic response [18] . Using CNPs instead of a cerium oxide support increases by two orders of magnitude the activity of a Au catalyst for the selective oxidation of CO [19] . In addition, the higher reactivity of CNPs at ambient temperatures is permitting many important biomedical applications to be developed, such as scavenging of reactive oxygen species (ROS) [12] , [20] , [21] , [22] . The CNP activity and toxicity to living tissue clearly depend on particle size and surface composition (e.g., Ce 3+ /Ce 4+ ratios), but as is normally the case in all areas of nanoparticle science, the problems of polydispersity, agglomeration, and surface variations have plagued detailed study of these parameters [10] , [23] , [24] . For CNPs, it is particularly challenging to determine the concentration and locations of Ce 3+ , attendant O vacancies, and protonated O (i.e., OH − , H 2 O) species on the surface, and the relationship between them [10] . A more controlled approach to monodisperse CeO 2 nanoclusters and nanoparticles is clearly needed, especially at the ultra-small, sub-20 nm sizes that are of growing importance, particularly for biomedical applications. We now describe development of procedures using simple Ce 4+ salts and organic reagents that yield a family of monodisperse ceria nanoclusters of different sizes depending on the carboxylic acid employed. Such an approach was recently accomplished for monodisperse metal nanoclusters, primarily of Au, stabilized by thiolate ligands [25] , [26] . In our work, the ligands of choice for metal oxide nanoclusters are carboxylates, especially since oleic and similar acids are common surfactants in metal oxide nanoparticle syntheses [20] , [27] . The solubility and monodisperse nature of the products we obtain allows molecular crystals to be grown, leading to structural characterization of the nanoclusters and their surface features to atomic precision by single-crystal X-ray diffractometry. The nanoclusters are [Ce 24 O 28 (OH) 8 (PhCO 2 ) 30 (py) 4 ] ( 1 ; Ce 24 ), [Ce 38 O 54 (OH) 8 (EtCO 2 ) 36 (py) 8 ] ( 2 ; Ce 38 ) and [Ce 40 O 56 (OH) 2 (MeCO 2 ) 44 (MeCO 2 H) 2 (py) 4 ]/[Ce 40 O 56 (OH) 2 (MeCO 2 ) 44 (MeCN) 2 (py) 4 ] ( 3a/b ; Ce 40 ), where py is pyridine. 3a / 3b denote the two independent nanoclusters in the asymmetric unit of 3 , which differ slightly in the organic ligation. 2 also contains two independent nanoclusters ( 2a / 2b ), but they have the same formulation. Nanocluster structures Several pertinent points about the complete structures of 1 – 3 (Fig. 1a –c) will be summarized to allow for convenient comparisons. They all comprise Ce x O y cores (excluding carboxylate O atoms) with metal ( x ) and total ( x + y ) atom counts of 24/60, 38/100 and 40/98 for 1 – 3 , respectively, and they exhibit the same fluorite structure as bulk CeO 2 , i.e., alternating layers of 8-coordinate cubic Ce 4+ and 4-coordinate tetrahedral O 2− ions. Some surface Ce 4+ ions are 7- or 9-coordinate (vide infra). From the viewpoint of Fig. 1d–f , the cores consist of five Ce layers in an A:B:C:B:A pattern ( 1 , A = 2, B = 6, C = 8; 2 , A = 4, B = 9, C = 12; 3 , A = 4, B = 10, C = 12), leading to the Ce 38 core of 2 being essentially spherical (1.12 × 1.12 × 1.12 nm) whereas those of Ce 24 ( 1 , 0.75 × 1.10 × 1.10 nm) and Ce 40 ( 3 , 1.13 × 1.13 × 1.61 nm) are ellipsoidal. The Ce 38 can also be described as a ‘truncated octahedron’, a structure that is one of those recently predicted by DFT studies to be favoured for Ce x O y fragments of CeO 2 in this size range [28] . 2 contains only Ce 4+ , but 1 and 3 each also contain two 10-coordinate Ce 3+ ions at opposite ends of the cores, as suggested by DFT calculations on Ce 3+ in Ce x O y fragments of CeO 2 [28] , [29] . The Ce oxidation states were confirmed by bond valence sum (BVS) calculations (Supplementary Table 2 ) and the detection of Ce 3+ ( S = ½) EPR spectra for 1 and 3 . 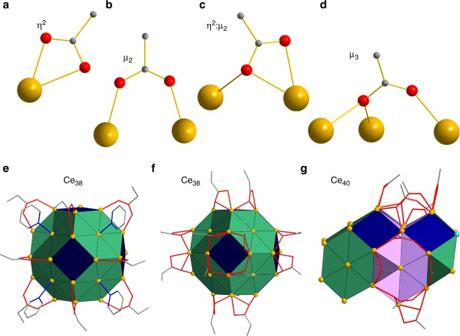Fig. 2 Ligand binding modes on the surface of ceria nanoclusters. The different binding modes of surface carboxylate and pyridine groups in1–3:achelating (η2);bµ2-bridging;cη2-chelating and µ2-bridging;dµ3-bridging;eCe38(2) showing terminal pyridines ‘capping’ (binding to the center of) the (111) hexagons, and µ2-carboxylates bridging edges joining two (111) facets;fCe38(2) showingη2:μ2-carboxylates at edges joining (100) and (111) facets; andgCe40(3) showingη2:μ2- and μ3-carboxylates on edges of (110) facets, and µ2-carboxylates bridging edges joining (110) and (111) facets. Colour code: CeIVgold, CeIIIsky-blue, O red, N blue, C grey, (100) facets dark blue; (110) facets violet; (111) facets green The latter were measured on microcrystalline powders at 5 K (Supplementary Figs. 1 and 2 ) and are comparable with the few Ce 3+ EPR spectra reported for CeO 2 nanoparticles or Ce 3+ doped into polymeric species [30] , [31] , [32] . Nanoclusters 1 – 3 are large enough to display multiple facets (Fig. 1g–i ), as do CNPs; the different faces for CeO 2 and Ce 40 are defined in Supplementary Fig. 3 . 1 and 2 display only (100) and (111) facets, whereas 3 exhibits these and also (110) facets. Finally, the cores are enveloped within monolayer organic shells of carboxylate and py groups, which exhibit only minor positional disorder in some C and O atoms (Fig. 1a–c ). Fig. 1 Structures of ceria nanoclusters. a – c show the complete structures of 1 (Ce 24 ), 2 (Ce 38 ), and 3a (Ce 40 ), respectively. H atoms have been omitted for clarity. Atom sizes of C, N, and O are made small to emphasize Ce locations. Colour code: Ce IV gold, Ce III sky blue, O red, N blue, C grey. d – f show their Ce/O cores from the same viewpoint (including carboxylate O atoms that are bridging) using the same colour code except that protonated O atoms (i.e., OH − ions) are indicated in purple. g – i show the cores again, from approximately the same viewpoint but with surface facets colour-coded: (100) facets are blue; (110) facets are violet; (111) facets are green. Only carboxylate O atoms that are bridging are included Full size image The structural results thus strongly support the description of 1 – 3 as atomically precise ceria nanoclusters in the ultra-small size range corresponding to the smallest CNPs synthesized to date, and stabilized to agglomeration by the organic monolayers. CNPs at this sub-20 nm size are being heavily targeted for use in various applications, especially in the biomedical field because they show enhanced catalytic activity and regenerative properties [21] , [33] , [34] . 1 – 3 are larger than the few previously known Ce/O molecular species, most of which are Ce 6 species [35] , [36] and some with tridentate amino-alcohol N,O,O-chelates [37] . It should be noted that the large family of monodisperse, crystalline polyoxometalates, some with very high metal nuclearities and sizes approaching 4 nm, have been known for many decades, but they do not possess the structure of bulk metal oxides and therefore cannot be described as their nanoparticles. Surface features X-ray crystallography has allowed definition to atomic resolution of the surfaces, which are crucial to CNP reactivity. The overall question is how the geometry and environments of surface Ce and O atoms differ from those of body atoms. Indeed, surface Ce 4+ geometries in 1 – 3 differ markedly from the 8-coordinate cubic of body Ce 4+ ions. Even those still 8-coordinate are significantly distorted, while many are 9-coordinate and there is even rare 7-coordination for Ce12/Ce22 in 3a/3b , respectively; coordination numbers are listed for all Ce atoms in Supplementary Table 2 . This variety reflects both the greater degrees of freedom at the surface and at the carboxylate ligation. Nevertheless, all body and surface Ce atoms are essentially at the positions they would occupy in bulk CeO 2 , as shown by the overlays in Supplementary Fig. 4 . The larger nanoclusters Ce 38 ( 2 ) and Ce 40 ( 3 ) show very little deviation of Ce and O atoms from their positions in bulk ceria; the smallest, Ce 24 ( 1 ), appears more pliable by showing greater deviation, but it is still small. Thus, the Ce x O y cores of 1 – 3 really can be described as fragments of bulk ceria, stabilized/passivated by the monolayer of carboxylate and pyridine ligands. There are four types of carboxylate binding in 1 – 3 (Fig. 2a–d ): chelating ( η 2 ) and three doubly or triply bridging modes, allowing for flexibility and versatility in binding to one, two, or V-shaped sets of three surface Ce ions. The carboxylates can thus accommodate the multi-faceted surface structure, including points of high curvature (Supplementary Fig. 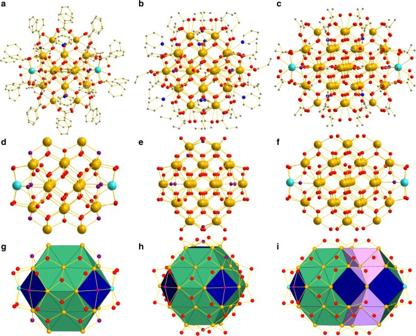5 ), with terminal py groups completing ligation where necessary. Fig. 1 Structures of ceria nanoclusters.a–cshow the complete structures of1(Ce24),2(Ce38), and3a(Ce40), respectively. H atoms have been omitted for clarity. Atom sizes of C, N, and O are made small to emphasize Ce locations. Colour code: CeIVgold, CeIIIsky blue, O red, N blue, C grey.d–fshow their Ce/O cores from the same viewpoint (including carboxylate O atoms that are bridging) using the same colour code except that protonated O atoms (i.e., OH−ions) are indicated in purple.g–ishow the cores again, from approximately the same viewpoint but with surface facets colour-coded: (100) facets are blue; (110) facets are violet; (111) facets are green. Only carboxylate O atoms that are bridging are included Both types of μ 2 -carboxylates occur in all three nanoclusters and bridge Ce 2 edges joining two facets, one of which is always a (111) facet (Table 1 and Fig. 2e–g ). Interestingly, the η 2 :μ 2 mode is found only at (100)(111) and (110)(111) edges, whereas the μ 2 mode is found only at (111)(111) and (110)(111) edges. In contrast, μ 3 -carboxylates occur only in 3 , bridging a V-shaped edge of the (110) facets. The η 2 -chelating mode is also only found in 3 , always bound to one Ce of a (100) Ce 4 square (vide infra). Terminal py ligands occur in all three nanoclusters, always ‘capping’ a (111) hexagon, i.e., attached to its central Ce (Fig. 2e ). The two independent Ce 38 nanoclusters in 2 are identical in formula and structure, but the two Ce 40 units in 3 provide the benefit of slightly differing organic monolayer shells, revealing one way the latter can vary for a given nanocluster core. Thus, the chelating carboxylates (Fig. 2a ) on two Ce 4+ ions (Ce9) in 3a are each replaced by a terminal MeCN (on Ce32) in 3b , converting 9-coordinate Ce9 into 8-coordinate Ce32. Fig. 2 Ligand binding modes on the surface of ceria nanoclusters. The different binding modes of surface carboxylate and pyridine groups in 1 – 3 : a chelating ( η 2 ); b µ 2 -bridging; c η 2 -chelating and µ 2 -bridging; d µ 3 -bridging; e Ce 38 ( 2 ) showing terminal pyridines ‘capping’ (binding to the center of) the (111) hexagons, and µ 2 -carboxylates bridging edges joining two (111) facets; f Ce 38 ( 2 ) showing η 2 :μ 2 -carboxylates at edges joining (100) and (111) facets; and g Ce 40 ( 3 ) showing η 2 :μ 2 - and μ 3 -carboxylates on edges of (110) facets, and µ 2 -carboxylates bridging edges joining (110) and (111) facets. Colour code: Ce IV gold, Ce III sky-blue, O red, N blue, C grey, (100) facets dark blue; (110) facets violet; (111) facets green Full size image Table 1 Type of surface ligands in nanoclusters 1–3 Full size table There are two distinct Ce surface subunits in 1 – 3 resulting from the fluorite structure, Ce 3 triangles and Ce 4 squares, and these will be described in turn. Ce 3 triangles are very common surface units in (111) and (110) facets and are bridged primarily by pyramidal μ 3 -O 2- ions (Table 1 ), from tetrahedral body O 2− ions now binding one less Ce. Some in 1 and 2 are instead bridged by μ 3 -OH − ions (Fig. 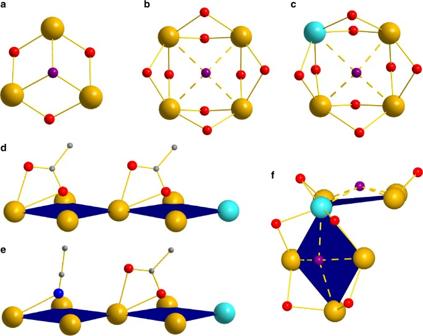Fig. 3 Structural features on the surface of ceria nanoclusters.aμ3-OH−on (111) CeIV3triangle;bμ4-OH−on a (100) CeIV4square;cμ4-OH−on a (100) CeIIICeIV3square;dη2-carboxylates in3aacting as lids on adjacent (100) CeIV4and CeIIICeIV3squares;ethe analogous situation in3bto that ind, with an MeCN ligand replacing oneη2-carboxylate as lid; andfμ4-OH−lids on a V-shaped (100) CeIIICeIV3double-square in1linked at the CeIIIcorner. Color code: CeIVgold, CeIIIsky-blue, O red, OH−purple, N blue, C grey. H atoms have been omitted for clarity 3a ): The four in 1 are obvious from their O-H···N hydrogen bonding to lattice py molecules (O···N = 2.7–2.9 Å), which thus anchors the H + on O15 and O16 and gives the expected O BVS of 1.21 (Supplementary Table 3 ). In contrast, the two μ 3 -OH − in 2 are disordered since there is no reason for H + to favour particular μ 3 -O 2− ions when so many are essentially equivalent. Slightly lowered BVS values (1.52–1.72) for the four μ 3 -O 2− ions at O18/O39 and the four at O49/O60 in 2a and 2b , respectively (Supplementary Table 4 ), suggest that the 2H + are randomly distributed primarily among these positions to give partial μ 3 -OH − occupancies. Fig. 3 Structural features on the surface of ceria nanoclusters. a μ 3 -OH − on (111) Ce IV 3 triangle; b μ 4 -OH − on a (100) Ce IV 4 square; c μ 4 -OH − on a (100) Ce III Ce IV 3 square; d η 2 -carboxylates in 3a acting as lids on adjacent (100) Ce IV 4 and Ce III Ce IV 3 squares; e the analogous situation in 3b to that in d , with an MeCN ligand replacing one η 2 -carboxylate as lid; and f μ 4 -OH − lids on a V-shaped (100) Ce III Ce IV 3 double-square in 1 linked at the Ce III corner. Color code: Ce IV gold, Ce III sky-blue, O red, OH − purple, N blue, C grey. H atoms have been omitted for clarity Full size image In body Ce 4 squares, each edge is oxide-bridged, but at the surface the edges are carboxylate-bridged. These are the (100) facets (Fig. 1g–i ) and occur in three slightly different forms. The six separated Ce 4+ 4 squares in 2 (Fig. 3b ), the two Ce 4+ 3 Ce 3+ Ce 4+ 3 V-shaped double-squares fused at a Ce 3+ corner in 1 (Fig. 3f ), and two Ce 4+ 3 Ce 3+ squares in 3 (Fig. 3c ) are all bridged by a μ 4 -OH − ion with rare tetragonal pyramidal geometry (the O is 0.7–0.8 Å above the Ce 4 plane). All μ 4 -OH − ions have similar O BVS values of 0.52–0.71 (Supplementary Tables 3 – 5 ), intermediate between those of OH − and H 2 O. In 1 (but not 2 or 3 ), the μ 4 -OH − protons (H12 and H14) were observed in difference Fourier maps, confirming them (and by extension those in 2 and 3 ) to be OH − , not H 2 O. The Ce 4+ ··OH − and Ce 3+ ··OH − distances are extremely long (2.7–3.0 Å; Supplementary Table 7 ) and suggest minimal Ce-O bonding; for comparison, Ce 4+ -μ 3 -O 2− = 2.2–2.3 Å, Ce 4+ -μ 4 -O 2− = 2.3–2.35 Å, and Ce 4+ -μ 3 -OH − = 2.3–2.45 Å. The very-long Ce··μ 4 -OH − distances suggest an essentially free OH − ion acting as a weakly docked ‘lid’ on the Ce 4 surface (and thus rationalizing its small BVS). Space-filling representations (Supplementary Fig. 6 ) show the OH − to be encapsulated by the surrounding carboxylates and cannot move from its μ 4 central position to become more strongly bound μ 2 or μ 3 . 3 also contains planar double-square units (Fig. 3d, e ), and these do not contain μ 4 -OH − ions. Instead, those in 3a (Fig. 3d ) have η 2 -carboxylates attached to one Ce that act as lids, tilting inwards so that one O atom approaches the mid-point of each square; the three resulting Ce··O separations (~3.0 Å) indicate extremely weak contacts (Supplementary Table 8 ). In 3b , one η 2 -carboxylate of each double-square is replaced by an MeCN, as described above, and this again tilts over the center of the square to act as a lid, giving a very unusual bent binding mode. The three resulting Ce··N separations (>3.0 Å) again indicate only very weak contacts. Interestingly, these planar double squares in 3 are each fused at their Ce 3+ corners to the μ 4 -OH − -bridged Ce 4+ 3 Ce 3+ squares (Fig. 3c ) described above, so that 3 contains two asymmetric L-shaped (86.1°) triple squares with the Ce 3+ lying at the inner point of the L. For charge balance, 3a must also contain two additional H + . Since the O BVS values indicate they are not on surface μ 3 -O 2− ions, we suspected them to be on ligand groups. Indeed, three carboxylate O atoms attached to Ce 3+ , namely O40, O40′ and O83, form a triangle and all show lowered BVS values of 1.78, 1.78 and 1.65, respectively, suggesting an H + is capping each of the two triangles in 3a by interacting with the O atoms in a trifurcated fashion (Supplementary Table 5 ). The formulation of 3b can now be rationalized as resulting from loss of some of the chelating MeCO 2 − groups in 3a , assisted by protonation to MeCO 2 H by these H + , and replacement by MeCN solvent molecules in 3b . The two Ce 3+ each in 1 and 3 are thus all at surface sites, as suggested to also be the case in CNPs [10] , [38] . The lower Ce 3+ charge favors fewer O 2− ligands than Ce 4+ and thus disfavors body sites. In contrast, 2 contains no Ce 3+ . Interestingly, all Ce 3+ occur within (100) Ce 4+ 3 Ce 3+ square facets. In 3 (Fig. 3c ), the Ce 3+ ··OH − and Ce 4+ ··OH − distances are identical (~2.7 Å), again supporting weak contacts by the μ 4 -OH − . In 1 , the V-shaped double-square joined at the Ce 3+ corner (Fig. 3f ) has a Ce 3+ ··OH − distance of ~ 2.7 Å on one side, but this causes a longer Ce 3+ ··OH − on the other (~3.0 Å; Supplementary Table 7 ). It is also extremely interesting that when Ce 3+ ions are present, the surface H + (i.e., OH − ions, and H + hydrogen bonding to carboxylate groups) are located very close to them. The presence and positions of H + on nanoparticles are extremely challenging to determine [39] , but in nanoclusters 1 and 3 most of them are directly observed and clearly accumulate on O atoms near Ce 3+ (Fig. 1d, f ). The effect is likely synergistic, i.e., the lower Ce 3+ charge favors accumulation of H + nearby, which in turn mollify the O 2− and carboxylate charges and stabilize the lower Ce 3+ charge. In contrast, with no Ce 3+ in 2 , the H + spread out over the surface (Fig. 1e ), although they again favor Ce 4 squares. H + are expected to be mobile on the nanocluster surfaces, as recent work has concluded from studies of hydrogen mobility (‘hopping’) on surface O atoms of CeO 2 thin films [40] . Double protonation of an O 2− and desorption of surface H 2 O was suggested as the means of forming O vacancies. We have shown that a bottom-up synthetic approach in solution at ambient temperatures using readily available reagents can be successfully applied to obtain a family of monodisperse metal oxide nanoparticles of ultra-small dimensions. This thus achieves for metal oxides what was previously accomplished for the distinctly different area of metal nanoparticles, particularly of Au. In the present work, monodisperse CeO 2 nanoclusters with the fluorite structure and monolayer organic ligand shells can be synthesized and structurally characterized to atomic resolution. They exhibit multifaceted structures consisting mainly of (100) and (111) facets, but 3 also has (110) facets giving noticeable surface kinks/edges/trenches. The surface location of any Ce 3+ ions and the H + positions on μ 3 - and μ 4 -OH − groups, as well as ligand groups, are particularly welcome to know. The μ 4 -OH − are weakly attached with long Ce···O distances to the (100) facets, acting as lids on Ce 4 squares, as also do O (carboxylate) and N (MeCN) lids on other (100) facets. Such surface features are likely of great relevance to CNP reactivity: Under heterogeneous catalysis conditions, or in solution or colloidal suspension, one can envisage the ready loss or ‘opening’ of such weakly interacting lids (e.g., by protonation of OH − , detachment of MeCN, or tilting away of the chelating carboxylate, perhaps by becoming monodentate) exposing Ce 4 square faces for reaction. We thus propose these weakly lidded Ce 4 sites as resting states of some of the catalytically highly reactive, surface O-vacancy sites in CNPs. In addition, when Ce 3+ ions are present, their locations in 1 and 3 corner-linking two (100) Ce 3+ Ce 4+ 3 squares, and the concomitant accumulation nearby of mobile H + , on μ 3 -OH − , μ 4 -OH − and/or ligand groups, together offer a possible picture for the high catalytic activity of surface Ce 3+ in CNPs. Similarly, the kinks/edges/trenches associated with the (110) facets in 3 suggest additional sites of increased reactivity, as seen for (110) facets of CNPs, and they have also been identified in CNPs as nucleation sites for heterometals [41] , [42] , a process we are trying to mimic with 3 . We note that there is a general consensus that the (111) facet of CNPs is the most thermodynamically stable while the (100) facet is highly reactive due its lower stability and is therefore a proposed site for O vacancies and Ce 3+ ions [17] , [29] , [43] , observations that are consistent with the surface features we have identified in 1 – 3 . Even on the basis of only the three nanoclusters described herein, it is already apparent how CNPs with similar sizes can have very different properties and reactivities. Although 2 and 3 are essentially the same size and metal nuclearity, they differ significantly in their overall shape, the variety of facets they exhibit, the resulting surface morphology, and their Ce 3+ content. On the other hand, the availability now of samples of identical, monodisperse nanoclusters makes possible the study of activity vs. exact size, surface morphology and Ce 3+ content. In addition, while dispersions of CNPs in water are often unstable, leading to agglomeration that can affect their transport, distribution and reactivity, particularly for ultra-small CNPs in biomedical studies, 3 is completely water soluble and affords the opportunity to study reactivity in biologically relevant media [27] , [44] . Finally, 1 – 3 contain either Ce 4+ 4 -μ 4 -OH − or Ce 3+ Ce 4+ 3 -μ 4 -OH − (100) squares, or both, and this variation may also be responsible for the recognized redox-state dependent ROS-scavenging ability and toxicity of CNPs with different amounts of surface Ce 3+ [21] , [22] , [45] , [46] . In contrast, recent suggestions that 1.1–3.5 nm CNPs should have a defect-fluorite structure and a large surface Ce 3+ :Ce 4+ ratio are not supported by 1 – 3 [47] , [48] . Ce 3+ is certainly on the surface, but no correlation between size and the number of Ce 3+ is seen, with Ce 24 and Ce 40 having two each, but Ce 38 none. In fact, given that Ce 3+ ions in 1 – 3 always occur at the centre of V-shaped double-square subunits (Fig. 3f and similar), we hypothesize that the higher symmetry, essentially spherical 2 contains no Ce 3+ because its surface structure contains no such double squares. Furthermore, the conventional wisdom that smaller CNPs have more surface Ce 3+ may reflect the greater number of such V-shaped units present in smaller nanoparticles of lower symmetry as a result of their increased number of points of high curvature. We are currently seeking to extend the family to larger nanoclusters and higher Ce 3+ :Ce 4+ ratios, and exploring the reactivity of 1 – 3 with ROS. Syntheses [Ce 24 O 28 (OH) 8 (PhCO 2 ) 30 (py) 4 ] ( 1 ) was prepared by the reaction of (NH 4 ) 2 [Ce(NO 3 ) 6 ] and PhCO 2 H in a 1:2 molar ratio in pyridine at room temperature. The golden-yellow solution was stirred for 30 mins, diluted with 2 volumes of MeCN, and maintained undisturbed for 1 week. The resulting yellow square plates of 1 ∙9py were collected by filtration, washed with MeCN, and dried in vacuum. The yield was 14% based on Ce. Anal. Calcd (Found) for dried 1 ∙2py (C 240 H 188 Ce 24 N 6 O 96 ): C, 35.79 (35.63); H, 2.35 (2.00); N, 1.04 (0.98). [Ce 38 O 54 (OH) 8 (EtCO 2 ) 36 (py) 8 ] ( 2 ) and[Ce 40 O 56 (OH) 2 (MeCO 2 ) 44 (MeCO 2 H) 2 (py) 4 ]/ [Ce 40 O 56 (OH) 2 (MeCO 2 ) 44 (MeCN) 2 (py) 4 ]( 3 ) were prepared by the reactionof (NH 4 ) 2 [Ce(NO 3 ) 6 ], the corresponding RCO 2 H, and NH 4 I in a 1:4:1 molar ratio in pyridine/H 2 O (10:1 v/v) at room temperature. The golden-yellow solutions were stirred for 30 min, diluted with two volumes of MeCN, and maintained undisturbed for 4 weeks. The resulting yellow square plates ( 2 ∙16MeCN) or rods ( 3 ∙48MeCN) were collected by filtration, washed with MeCN, and dried in vacuum. The yields were 49% and 35% for 2 and 3 , respectively. Anal. Calcd (Found) for 2 ∙7H 2 O (C 148 H 242 Ce 38 N 8 O 141 ): C, 18.30 (17.90); H, 2.51 (2.36); N, 1.15 (1.05). Anal. Calcd (Found) for 3∙ 8H 2 O (C 112 H 178 Ce 40 N 5 O 156 ): C, 13.88(13.79); H, 1.85 (1.78); N, 0.72 (0.76). The indicated atomic composition of 3 is calculated using the average of the 3a and 3b formulas. Fuller details of the three syntheses and infra-red spectral data for 1 – 3 are available in Supplementary Methods . X-ray crystallography Single-crystal X-ray diffraction studies at −173 °C were performed on a Bruker DUO diffractometer using MoK α ( λ = 0.71073 Å) or CuK α ( λ = 1.54178 Å) radiation (from an ImuS power source), and an APEXII CCD area detector ( Supplementary Methods and Supplementary Table 1 ). The metric parameters of the refined structures were used to determine the Ce oxidation states and the O protonation levels by bond valence sum (BVS) calculations (Supplementary Tables 2 – 5 ). Data availability The crystallographic information files (CIFs) for [Ce 24 O 28 (OH) 8 (PhCO 2 ) 30 (py) 4 ]∙9py ( 1 ∙9py), [Ce 38 O 54 (OH) 8 (EtCO 2 ) 36 (py) 8 ]∙16MeCN ( 2 ∙16MeCN), and [Ce 40 O 56 (OH) 2 (MeCO 2 ) 44 (MeCO 2 H) 2/0 (MeCN) 0/2 (py) 4 ]∙48MeCN ( 3 ∙48MeCN) have been deposited at the Cambridge Crystallographic Data Centre with deposition codes CCDC 1529955-1529957 for 1 – 3 , respectively.